Information flow through neural circuits for pheromone orientation Moths use a sophisticated olfactory navigation strategy for resource localization. Here we investigate the neuronal circuits involved in sensory processing to generate locomotor commands for pheromone-source orientation in the moth. We identify a candidate pathway for pheromone processing in the protocerebrum using a mass-staining technique. Our intracellular recordings of pheromone responsiveness detect four major circuits, including a newly identified unstructured neuropil, the superior medial protocerebrum, which supplies output to the lateral accessory lobe (LAL), the premotor centre for walking commands. Interneurons innervating the lower division of the LAL elicited longer responses than those innervating the upper division. Descending interneurons innervating the lower division of the LAL showed a state-dependent flip-flop response. In contrast, input from other visual areas in the protocerebrum mostly converge onto the upper division of the LAL. These results reveal the basic organization of the LAL: the upper division is identified as a protocerebral hub that receives inputs from various areas, while the lower division generates long-lasting activity for locomotor command. Animals use a sophisticated navigation strategy to respond to olfactory signals, which are crucial for finding food, mating partners and predators. Male moths orient themselves towards conspecific females in response to sex pheromones by two patterns of locomotion: an initial surge and zig-zag casting behaviour [1] , [2] , [3] . Zig-zag locomotion has been reported in a wide range of animal species comprising of insects [4] , [5] and mammals [6] , including humans [7] . In moths, sex pheromones have been shown to reliably elicit stereotyped behaviour and, hence, can be used as a good model for investigating the general mechanisms underlying olfactory navigation. In the moth brain, sex pheromones are first processed by the primary olfactory centre, the antennal lobe (AL), in which the spatio-temporal features of the stimulus are extracted [8] , [9] . Projection neurons receive an input from the macroglomerular complex (MGC) in the AL, and subsequently convey the processed information into the lateral protocerebrum [10] . The lateral accessory lobe (LAL) receives processed information via an unknown area in the protocerebrum, and functions as a premotor circuit for pheromone orientation [11] , [12] . Descending interneurons (DNs) link the brain and ventral nerve cord. DNs innervating the LAL exhibit characteristic state-dependent long-lasting firing activity, which has been correlated with locomotion during orientation behaviour to the pheromone source [13] , [14] . The descending pathway through the LAL has also been identified in other insect taxa [15] , [16] , [17] , [18] . Although pheromone-responsive neurons in the protocerebrum have been reported in moths [11] , [19] , [20] , the neurons mediating the pathway from the sensory area to the premotor centre remain largely unknown. Since sex pheromones reliably induce stereotypic behavioural output, the connection may exist between the primary olfactory centre and premotor area. The protocerebrum has a lot of terra incognita . The traditional blind intracellular recording technique alone is not feasible for examining information flow in the brain. We used mass staining of a population of neurons and constructed a wiring diagram for brain regions in the protocerebrum of the silkmoth Bombyx mori . On the basis of this areal connectivity, we then obtained single-cell recordings from the region of interest to search previously unknown pathways. This combination enabled us to compare neuronal responses at each stage of processing. The neural pathway for pheromone processing The AL and LAL are highly associated with pheromone processing [14] , [21] . The delta area of the inferior lateral protocerebrum (ΔILPC) has also been identified as the second order centre [10] . However, connectivity between the ΔILPC and LAL remains unknown. To identify the pathway involved in pheromone processing, we first examined brain-wide areal connectivity using mass staining ( Figs 1 and 2 ) in combination with intracellular recording and staining techniques ( Fig. 3 ). Mass staining by injecting dyes into the ΔILPC labelled a maximum of 163 cells in 8 different cell clusters ( n =5 samples; Figs 1c–h and 2a ). The superior medial protocerebrum (SMP) was densely labelled in both hemispheres ( Fig. 1c,e,f ), which indicates that this area is connected to the ΔILPC. The toroid glomerulus, which processes bombykol, the primary pheromone component of B. mori in the ipsilateral MGC, was also labelled ( Fig. 1d ; Supplementary Fig. 1 ) and its morphology was consistent with the projection neurons innervating the toroid [21] . Two types of neurons connected the ΔILPC to the SMP: neurons connecting the ΔILPC and SMP in both hemispheres ( Fig. 3d ) and neurons connecting the ΔILPC and SMP in the ipsilateral hemisphere ( Supplementary Fig. 2a ). Cell bodies were located in the area surrounding the calyx of the mushroom body (MB), in which a group of neurons that exhibit neural activity in response to the sex pheromone are present [22] . All neurons with smooth processes, which is an indicator of a postsynaptic terminal [23] , within the ΔILPC showed a transient excitatory response to bombykol on both the ipsi- and contralateral sides ( n =5 neurons, Fig. 3d,e,h,i ; Supplementary Fig. 2 for morphology). Projection neurons innervating the toroid did not respond to stimulation of the contralateral antenna ( n =6 neurons; Fig. 3b,c,h ), which indicates that bilateral information is initially integrated at the level of the ΔILPC, the second order centre. 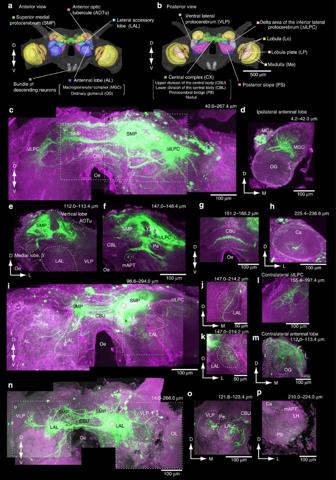Figure 1: Areal connectivity involved in pheromone processing as estimated by mass staining of the neuronal population. (a,b) Anterior and posterior views of the brain of the silkmoth. Major neuropils are labelled by colour. (c) Mass staining by injecting dye in the ΔILPC. The ipsilateral AL (d), ipsi- and contralateral SMP (e,f), contralateral ΔILPC, CBU (upper division of the central body) (g) and ipsilateral calyx of the mushroom body (h) were labelled. Micrographs ofc–hare from the same preparation. (i) Mass staining by injecting dye in the SMP. The contralateral SMP, ipsi- and contralateral LAL (j,k), contralateral ΔILPC (l), contralateral AL (m) and CBU were labelled. Micrographs ofi–mare from the same preparation. (n) Mass staining by injecting dye in the LAL. The ipsi- and contralateral SMP, contralateral LAL (o), ipsi- and contralateral VLP (n), CBU, ipsilateral optic lobe (OL) and ipsilateral PS (p) were labelled. Micrographs of (o–p) are from the same preparation. Ca, calyx of the mushroom body; LH, lateral horn; mAPT, medial antenno-protocerebral tract; MC, medial cell cluster of the AL; Oe, Oesophagus; Pe, pedunculus; Y, Y-tract. Figure 1: Areal connectivity involved in pheromone processing as estimated by mass staining of the neuronal population. ( a , b ) Anterior and posterior views of the brain of the silkmoth. Major neuropils are labelled by colour. ( c ) Mass staining by injecting dye in the ΔILPC. The ipsilateral AL ( d ), ipsi- and contralateral SMP ( e , f ), contralateral ΔILPC, CBU (upper division of the central body) ( g ) and ipsilateral calyx of the mushroom body ( h ) were labelled. Micrographs of c – h are from the same preparation. ( i ) Mass staining by injecting dye in the SMP. The contralateral SMP, ipsi- and contralateral LAL ( j , k ), contralateral ΔILPC ( l ), contralateral AL ( m ) and CBU were labelled. Micrographs of i – m are from the same preparation. ( n ) Mass staining by injecting dye in the LAL. The ipsi- and contralateral SMP, contralateral LAL ( o ), ipsi- and contralateral VLP ( n ), CBU, ipsilateral optic lobe (OL) and ipsilateral PS ( p ) were labelled. Micrographs of ( o – p ) are from the same preparation. Ca, calyx of the mushroom body; LH, lateral horn; mAPT, medial antenno-protocerebral tract; MC, medial cell cluster of the AL; Oe, Oesophagus; Pe, pedunculus; Y, Y-tract. 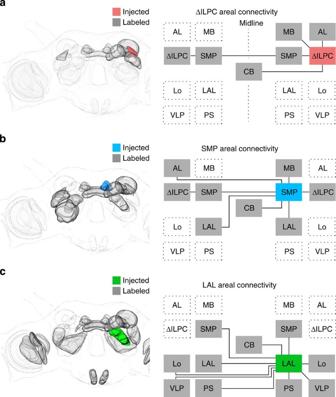Figure 2: Schematic diagram of mass-staining results. (a) Staining results for the dye injection to the ΔILPC. Reconstructed neuropils (left) and wiring diagram of the areal connectivity are shown (right). The coloured region represents the site of the dye injection and grey represents the labelled regions. (b) Staining results for the dye injection to the SMP. (c) Staining results for the dye injection to the LAL. Full size image Figure 2: Schematic diagram of mass-staining results. ( a ) Staining results for the dye injection to the ΔILPC. Reconstructed neuropils (left) and wiring diagram of the areal connectivity are shown (right). The coloured region represents the site of the dye injection and grey represents the labelled regions. ( b ) Staining results for the dye injection to the SMP. ( c ) Staining results for the dye injection to the LAL. 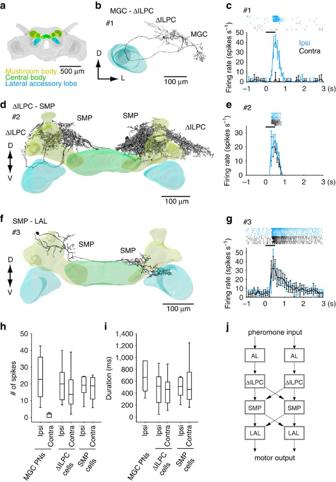Figure 3: Neurons constituting pheromone-processing circuits in the moth brain. (a) Major structured neuropils in the silkmoth brain. (b) Reconstruction of the antennal lobe projection neuron. (c) Physiology of the antennal lobe projection neuron shown inb, in response to the pheromone. Data are presented as the mean±s.d. (d) Reconstruction of the neuron innervating the delta area of the inferior lateral protocerebrum (ΔILPC) and superior medial protocerebrum (SMP) on both hemispheres. (e) Physiology of the ΔILPC cell is shown ind, in response to the pheromone. (f) Reconstruction of the neuron innervating SMP on both sides and contralateral LAL. (g) Physiology of the SMP cell is shown inf, in response to the pheromone. (h) Comparison of the firing-rate change of each neuron type in response to the ipsilateral and contralateral stimuli. The response of the antennal lobe projection neuron was significantly higher to the ipsilateral stimulation than to the contralateral stimulation (P=0.0313,n=6 neurons, Mann–WhitneyU-test). No significant difference was observed in the responses to the ipsilateral and contralateral stimuli for other neuron types (P=0.188,n=5 neurons for ΔILPC;P=0.054,n=8 neurons for SMP; Mann–WhitneyU-test). (i) Comparison of the response durations among each neuron type in response to the ipsilateral and contralateral stimuli. No significant difference was observed in the responses to the ipsilateral and contralateral stimuli for other neuron types. (j) The proposed pathway for pheromone processing in the silkmoth brain. Full size image Figure 3: Neurons constituting pheromone-processing circuits in the moth brain. ( a ) Major structured neuropils in the silkmoth brain. ( b ) Reconstruction of the antennal lobe projection neuron. ( c ) Physiology of the antennal lobe projection neuron shown in b , in response to the pheromone. Data are presented as the mean±s.d. ( d ) Reconstruction of the neuron innervating the delta area of the inferior lateral protocerebrum (ΔILPC) and superior medial protocerebrum (SMP) on both hemispheres. ( e ) Physiology of the ΔILPC cell is shown in d , in response to the pheromone. ( f ) Reconstruction of the neuron innervating SMP on both sides and contralateral LAL. ( g ) Physiology of the SMP cell is shown in f , in response to the pheromone. ( h ) Comparison of the firing-rate change of each neuron type in response to the ipsilateral and contralateral stimuli. The response of the antennal lobe projection neuron was significantly higher to the ipsilateral stimulation than to the contralateral stimulation ( P =0.0313, n =6 neurons, Mann–Whitney U -test). No significant difference was observed in the responses to the ipsilateral and contralateral stimuli for other neuron types ( P =0.188, n =5 neurons for ΔILPC; P =0.054, n =8 neurons for SMP; Mann–Whitney U -test). ( i ) Comparison of the response durations among each neuron type in response to the ipsilateral and contralateral stimuli. No significant difference was observed in the responses to the ipsilateral and contralateral stimuli for other neuron types. ( j ) The proposed pathway for pheromone processing in the silkmoth brain. Full size image We also injected dyes into the lateral horn, in which the projection neurons innervating non-pheromonal glomeruli send axon terminals [10] , [24] ( Supplementary Fig. 3 ). The ipsilateral AL, calyx of the MB, superior lateral protocerebrum and contralateral lateral horn were densely labelled. The SMP was not labelled, indicating that the connection with SMP in the lateral protocerebrum is specific to the ΔILPC, which receives bombykol-specific information [10] , [21] . We then injected dyes into the SMP, and labelled a maximum of 241 cells in 9 cell clusters ( n =5 samples; Figs 1i–m and 2b ). The ΔILPC on both hemispheres, the contralateral SMP and the LAL on both hemispheres were labelled. All neurons with smooth processes with the SMP responded to the sex pheromone ( n =8 neurons, Fig. 3f–i ; Supplementary Fig. 4 ). Several neurons also innervated the upper division of the central body ( Fig. 1i ). The neurons connecting the SMP and central body were identified by intracellular staining ( Supplementary Fig. 5b for morphology). Neurons with smooth processes in the central body did not exhibit excitatory responses to the sex pheromone ( n =7 neurons; Supplementary Fig. 5 ); therefore, this pathway may have contributed less to pheromone processing compared with other regions. A few fibres connecting with AL were labelled ( Fig. 1m ). The neurons with a smooth process in the SMP and varicose process in the AL were identified by intracellular recording ( Supplementary Fig. 6 ). These neurons may mediate a putative feedback pathway from the SMP to AL because the innervations in the SMP were smooth, and those in the AL were mostly varicose, which is an indicator of a presynaptic terminal [23] . SMP neurons showed transient excitatory responses to bombykol, which were stronger than those to other plant odours ( Supplementary Fig. 7 ). These results suggest that SMP is the relay of the ΔILPC and LAL for sex pheromone processing; however, further investigations with stimuli of other sensory modalities are required. We further performed mass staining by injecting dyes into the LAL, and labelled a maximum of 110 cells in 12 different cell clusters ( n =42 samples; Figs 1n–p and 2c ). The contralateral LAL and SMP on both hemispheres were densely labelled, whereas no cells were labelled in the AL or ΔILPC. Mass staining revealed that LAL neurons also connected with the central complex (CX), including the central body and protocerebral bridge, ventrolateral protocerebrum (VLP), optic lobe (OL) and posterior slope (PS) ( Fig. 1n–p ). Neurons with smooth processes in the CX, VLP and OL did not exhibit excitatory responses to bombykol ( n =7 neurons for the CX ( Supplementary Fig. 5 ); n =7 neurons for the VLP ( Supplementary Fig. 8 ); n =19 neurons for the OL ( Supplementary Fig. 9 )), which suggest that these areas were not highly relevant for sex pheromone processing. In contrast, 6 out of a total of 10 neurons with smooth processes in the PS exhibited excitatory responses to bombykol ( Supplementary Fig. 10 ). We did not find the connection from the ΔILPC or SMP to the PS with either mass staining ( n =3 for dye injection into the PS; Supplementary Fig. 11 ) or single-cell labelling. Neurons that were sensitive to the sex pheromone were detected in other brain regions that were not labelled by mass staining (20% of neurons innervating the lateral horn ( n =5), 47.9% of the lateral protocerebrum other than the ΔILPC ( n =48) and 55.5% of the subesophageal ganglion ( n =9)). Long-lasting firing activity, which persists after termination of the stimulus, was not observed in any of the brain interneurons mentioned above. Two types of interneurons are known to innervate the LAL: unilateral neurons (UNs) innervating the LAL on one side and bilateral neurons (BNs) innervating the LAL on both sides ( Fig. 4a ) [25] . Eight out of a total of 20 stained BNs had varicose processes in the contralateral PS and five out of a total of nine stained UNs had varicose processes in the ipsilateral PS ( Supplementary Fig. 12 ; Supplementary Table 1 ). In addition to known UNs, we newly identified a novel type, which innervated both the LAL and anterior SMP (LAL–SMP UNs; Supplementary Fig. 13 ). Their cell bodies belonged to the cell cluster located anteriodorsally to the medial lobe of the MB. In contrast to the known UN type, the neurite of this LAL–SMP UN appeared to be axon-less and did not show any varicose process, as has been reported in local interneurons in the AL [10] . Most LAL–SMP UNs exhibited transient excitatory responses that lasted up to ~2,000 ms, which were similar to UNs without innervation in the SMP [25] . All UNs responded to the stimulation on both sides of the antennae ( Supplementary Fig. 13c ). These interneurons may also mediate information flow from the SMP to LAL for sex pheromone processing. 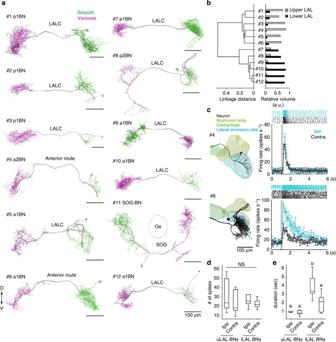Figure 4: Neurons innervating the lower LAL exhibited longer activity duration. (a) Morphology of the LAL bilateral neurons. The neuron types were noted based on the cell body position and neurite innervation25. The areas in which the majority of terminals showed smooth processes and varicose processes are shown with green and magenta, respectively. Cell body location of #12 is shown by an asterisk. (b) Clustering of LAL bilateral neurons based on the density of smooth processes (left). Relative volumes of the neurites of LAL bilateral neurons in the upper (grey) and lower divisions of the LAL (black) are shown (right). The number in the vertical axis corresponds to the numbers in columna. (c) Physiology of LAL bilateral neurons with the dendrite mainly in the upper division (top) and lower division of the LAL (bottom). Reconstructed morphology (left) and the response of corresponding cells are shown (right). Data are presented as the mean±s.d. (d) Comparison of the response amplitude. The firing rate change after the stimulus onset was calculated. No significant difference was observed in the responses of lower LAL-dominant BNs (lLAL BNs) and upper LAL-dominant BNs (uLAL BNs) (F(3, 20)=0.66,P=0.589,n=6, 6 neurons for lLAL BNs and uLAL BNs, one-way analysis of variance (ANOVA) followed by Scheffe’sF-test). (e) Comparison of response durations. The response duration to the ipsilateral stimulation of lLAL BNs was significantly longer than that of uLAL BNs. The response duration to the ipsilateral stimulation of lLAL BNs was significantly longer than that to the contralateral stimulation (P<0.005; one-way ANOVA followed by Scheffe’sF-test). LALC, lateral accessory lobe commissure. NS, not significant. Figure 4: Neurons innervating the lower LAL exhibited longer activity duration. ( a ) Morphology of the LAL bilateral neurons. The neuron types were noted based on the cell body position and neurite innervation [25] . The areas in which the majority of terminals showed smooth processes and varicose processes are shown with green and magenta, respectively. Cell body location of #12 is shown by an asterisk. ( b ) Clustering of LAL bilateral neurons based on the density of smooth processes (left). Relative volumes of the neurites of LAL bilateral neurons in the upper (grey) and lower divisions of the LAL (black) are shown (right). The number in the vertical axis corresponds to the numbers in column a . ( c ) Physiology of LAL bilateral neurons with the dendrite mainly in the upper division (top) and lower division of the LAL (bottom). Reconstructed morphology (left) and the response of corresponding cells are shown (right). Data are presented as the mean±s.d. ( d ) Comparison of the response amplitude. The firing rate change after the stimulus onset was calculated. No significant difference was observed in the responses of lower LAL-dominant BNs (lLAL BNs) and upper LAL-dominant BNs (uLAL BNs) (F(3, 20)=0.66, P =0.589, n =6, 6 neurons for lLAL BNs and uLAL BNs, one-way analysis of variance (ANOVA) followed by Scheffe’s F -test). ( e ) Comparison of response durations. The response duration to the ipsilateral stimulation of lLAL BNs was significantly longer than that of uLAL BNs. The response duration to the ipsilateral stimulation of lLAL BNs was significantly longer than that to the contralateral stimulation ( P <0.005; one-way ANOVA followed by Scheffe’s F -test). LALC, lateral accessory lobe commissure. NS, not significant. Full size image Modular organization of the LAL Insects steer upwind by using visual information, and visual feedback is important for upwind orientation in moths (optomotor anemotaxis) [26] . Even when domesticated, silkmoths utilize visual information to modify locomotor commands to adapt to perturbations in the sensory-motor feedback gain [27] , [28] . We next analysed the pathway from the visual neuropils onto the pheromone pathway identified in the present study. We found that interneurons supplied an input to the LAL from other visual areas in the protocerebrum ( Supplementary Fig. 5 for CX, Supplementary Fig. 9 for OL and Supplementary Fig. 14 for anterior optic tubercle (AOTu)). We stained 19 neurons that had smooth processes in the OL and projected to the protocerebrum. Neurons innervating the lobula complex (either from the lobula or lobula plate) also innervated the LAL as well as the PS, whereas neurons innervating the medulla mainly projected to the posterior part of the brain ( Supplementary Fig. 10h,i ) without innervation to the LAL. Some neurons from the lobula complex showed wide-field dendritic branches ( Supplementary Fig. 9a–d ), which is reminiscent of lobula plate tangential cells reported in the fly [29] . Neurons innervating the lobula complex did not show excitatory responses to bombykol, and the activity during light stimulation were slightly inhibited ( P =0.0079, Mann–Whitney U -test, n =5 neurons). There was a bias in the connectivity between the lobula complex and LAL. The LAL has been shown to have two subdivisions that are defined by the LAL commissure: upper and lower divisions [25] , corresponding to dorsal and ventral LAL in the butterfly based on anatomical features [30] . The volume of putative input processes was significantly larger in the upper LAL than in the lower LAL ( Supplementary Fig. 9j ; P =7.5 × 10 −9 , t 12 =14.2, n =13 neurons, paired t -test), which demonstrate that the upper division of the LAL was the output area of the lobula complex, which provides information on global visual motion. In addition, neurons from the CX preferentially innervated the upper division of the LAL ( Supplementary Fig. 5e ; P =9.9 × 10 −5 , t 4 =15.6, n =5 neurons, paired t -test). Similar biased innervations to the upper division were observed in neurons innervating the AOTu ( Supplementary Fig. 14 ). Thus, the upper division of the LAL connected strongly with other brain regions and was distinct from the lower division in terms of neuronal connectivity. These results revealed the presence of anatomically distinct modules in the LAL: input from the other part of the protocerebrum mostly converges onto the upper division. We then searched for functional differences in the upper and lower divisions of the LAL. LAL BNs have smooth branches, which are supposed to be an input area, in one side of the LAL [25] ( Fig. 4a , green). We performed a clustering analysis to determine the density of smooth processes among BNs ( Fig. 4b ) and classified them into two groups: the lower LAL-dominant type and upper LAL-dominant type. The lower LAL-dominant type of BNs, which have a larger neurite volume in the lower division showed longer responses to exposure to the sex pheromone ( Fig. 4c,e ; P <0.005, n =6 neurons for each type, one-way analysis of variance followed by Scheffe’s F -test). This differential response property indicates that the two anatomical modules, the upper and lower divisions of the LAL, may have different functions in pheromone processing. No significant differences were observed in response amplitudes ( Fig. 4d ). State-dependent activity in DNs Insects have several hundred DNs that connect the brain and ventral nerve cord [31] , [32] , [33] . We performed backfill labelling from the cut end of the neck connective, and the cell bodies of approximately half of the DNs were located in the supraesophageal ganglion ( Fig. 5a ). Of these, group-I and group-II DNs, the populations whose cell bodies are located in the anterior part of the brain ( Fig. 5a,b #1–4), contained DNs that innervated the LAL [34] . Eleven group-I DNs had varicose processes in the contralateral PS and five group-II DNs had varicose processes in the ipsilateral PS ( Fig. 5b ; Supplementary Fig. 12g,h ; Supplementary Table 1 ). Six out of a total of 15 group-I/II DNs exhibited characteristic state-dependent activity that resembled an electronic ‘flip-flop (FF) circuit’, which has two distinct firing frequencies ( Fig. 5c ) [13] . We found that the dendrites of these DNs mostly innervated the lower division of the LAL ( Supplementary Fig. 15 ), suggesting the importance of the lower division on the generation of FF signals. Once activated, these DNs exhibited a sustained firing activity that lasted >30 s. In a total of five group-III DNs, whose cell bodies were located in the posterior part of the brain ( Fig. 5a,b #5–8), three exhibited transient excitatory responses and did not have the long-lasting firing, which was observed in group-I/II DNs. The responses in five out of a total of six FF DNs showed bi-phasic dynamics: transient excitation in the early phase and sustained firing in the late phase of the response ( Fig. 5d , top, asterisk). The transition probability was independent of the firing rate in the early phase. Similar dynamics in neuronal activity have been reported previously in the pyramidal cells of the ferret prefrontal cortex [35] and rodent cerebellar Purkinje cells [36] . As in these cases, FF DNs showed bistability in their activity levels ( Fig. 5e ). Since the time course was similar to the responses observed in upstream neurons (that is, the ΔILPC and SMP cells), the responses of DNs in the early phase may mainly reflect a direct input from SMP to the LAL. Transient excitation was also observed in the transition from the ON to OFF state ( Fig. 5d , bottom, asterisk). Furthermore, transient inhibition was observed in failure trials of the ON to ON state ( Fig. 5c , middle), which suggests the existence of balanced excitatory and inhibitory inputs during state transition. 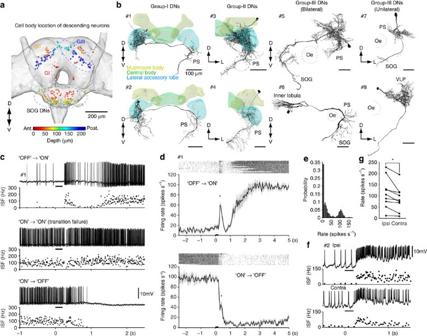Figure 5: Morphology and physiology of descending neurons. (a) Distribution of cell bodies in the descending neurons (DNs) stained by backfilling from the neck connective. The depth of the cell body position is shown by a pseudocolour. (b) Morphology of silkmoth DNs. Group-I DNs (#1, #2), group-II DNs (#3, #4) and group-III DNs (#5–#8) are shown. (c) Physiology of LAL DN (#1 inb) in response to the sex pheromone. Membrane potentials and instantaneous spike frequencies (ISFs) to three consecutive 200-ms stimuli are shown: transition from the ‘OFF’ to the ‘ON’ state (top), ‘ON’ to the ‘ON’ state (middle) and ‘ON’ to the ‘OFF’ state (bottom). (d) Firing-rate changes in the flip-flop response of LAL DN (#1 inb). Spike timing and mean firing-rate changes in response to the sex pheromone stimulation are shown. Data are presented as the mean±s.e.m. Through the transition in both cases of ‘OFF’ to ‘ON’ and ‘ON’ to ‘OFF’, brief transient excitation was observed (shown by asterisks). (e) Bistability of flip-flop DNs modulated by the pheromone stimulation (bin size 5 Hz). (f) Physiology of LAL DNs (#2 inb) in response to the pheromone stimulation on ipsilateral (top) and contralateral antennae (bottom). Membrane potentials and instantaneous spike frequencies are shown. (g) Firing rates were higher in response to the ipsilateral stimulation than to the contralateral stimulation (P=0.0039, Wilcoxon signed rank test,n=9 neurons). Figure 5: Morphology and physiology of descending neurons. ( a ) Distribution of cell bodies in the descending neurons (DNs) stained by backfilling from the neck connective. The depth of the cell body position is shown by a pseudocolour. ( b ) Morphology of silkmoth DNs. Group-I DNs (#1, #2), group-II DNs (#3, #4) and group-III DNs (#5–#8) are shown. ( c ) Physiology of LAL DN (#1 in b ) in response to the sex pheromone. Membrane potentials and instantaneous spike frequencies (ISFs) to three consecutive 200-ms stimuli are shown: transition from the ‘OFF’ to the ‘ON’ state (top), ‘ON’ to the ‘ON’ state (middle) and ‘ON’ to the ‘OFF’ state (bottom). ( d ) Firing-rate changes in the flip-flop response of LAL DN (#1 in b ). Spike timing and mean firing-rate changes in response to the sex pheromone stimulation are shown. Data are presented as the mean±s.e.m. Through the transition in both cases of ‘OFF’ to ‘ON’ and ‘ON’ to ‘OFF’, brief transient excitation was observed (shown by asterisks). ( e ) Bistability of flip-flop DNs modulated by the pheromone stimulation (bin size 5 Hz). ( f ) Physiology of LAL DNs (#2 in b ) in response to the pheromone stimulation on ipsilateral (top) and contralateral antennae (bottom). Membrane potentials and instantaneous spike frequencies are shown. ( g ) Firing rates were higher in response to the ipsilateral stimulation than to the contralateral stimulation ( P =0.0039, Wilcoxon signed rank test, n =9 neurons). Full size image The turning direction of initial walking for pheromone orientation was previously shown to be largely determined by the laterality of the pheromone input [37] . Moths exhibit turning behaviour towards the side of the pheromone input. Since FF DNs are thought to play a role in motor command, we measured differences between neural responses in the early phase, which roughly correspond to the time window for the initial surge direction. A surge was observed in male silkmoths ~300 ms after the stimulus onset and lasted ~0.5 s (ref. 38 ). Stimulation of the ipsilateral antennae induced higher firing activity than that of the contralateral antennae ( Fig. 5f,g ), which suggests that the difference between the left and right DN populations determine the initial walking direction. We characterized the pheromone responsiveness of neurons at each stage of the circuit. Among the brain regions examined, neurons with smooth branches in the MGC, ΔILPC, SMP and LAL showed excitatory responses to the sex pheromone. We identified a sensory-motor pathway for pheromone processing in the brain: a pheromone input was relayed in the MGC, ΔILPC, SMP and LAL to finally reach the DNs ( Fig. 3j ). A subpopulation of neurons innervating the PS also showed transient excitation to sex pheromone. Some DNs showing long-lasting firing, which is believed to be a locomotor command [13] , [14] , did not have smooth processes in the PS ( Fig. 5b : #3,4, Supplementary Table 1 ). This indicates that the PS is not necessary for state-dependent long-lasting firing. However, the PS may also contribute to locomotor control because the dense dendritic innervation of DNs was observed in this area ( Supplementary Fig. 16 ). We assume that the PS is a downstream of the LAL for the following two reasons: (i) Most of the interneurons connecting the LAL and PS had smooth processes in the LAL and varicose processes in the PS ( Fig. 5b ; Supplementary Fig. 12 ; Supplementary Table 1 ), (ii) PS did not have connections to the other circuits for pheromone processing. Mass staining by injecting dye into the ΔILPC and SMP did not label the PS ( Fig. 1 ), and the dye injection into the PS did not label ΔILPC or SMP ( Supplementary Fig. 11 ), suggesting that the PS receives pheromone information from the LAL. On the basis of individual neuronal morphologies ( Supplementary Fig. 4 ) and pheromone responsiveness ( Fig. 2 ), the SMP may provide an input onto both sides of the LAL. This organization is similar to the premotor centre in the lamprey, in which the activation of an upstream circuit on one side was shown to elicit similar synaptic inputs on both sides of the reticulospinal neurons, a counterpart of insect DNs [39] . In addition to the LAL, the SMP also supplied an input to the CX in the moth ( Fig. 1i ; Supplementary Fig. 5b ). CX neurons provided inputs to the upper division of the LAL ( Supplementary Fig. 5f ). Therefore, there are at least two pathways for the connection between the SMP and LAL: an indirect pathway through the CX [40] and a direct pathway described in the present study. Visual responses of the neurons innervating the CX and OL were suppressed by exposure to bombykol ( Supplementary Figs 5 and 9 ). The role of this inhibition currently remains unknown. One possibility is that the suppression observed was caused by corollary discharge, which enables animals to process self-generated sensory information compared with others perceived from their external environment [41] , [42] . The suppression of sensory signals has been reported in optomotor response during flight [43] and escape turns in the locust [44] , and auditory processing during song generation in crickets [45] . Sensory stimuli that should trigger behaviour may be able to cause suppression without actual behavioural output. For example, sensory stimuli used to elicit defensive kicking can sometimes suppress visual interneurons without the actual occurrence of kicking [46] . Similar to this case, we assume that the presence of an inhibitory feedback from premotor to sensory areas for corollary discharge in the moth. Moths always exhibit straight walking immediately after a pheromone input. Although moths were fixed during the recording, the signal from the LAL to OL may have suppressed the visual input to compensate for the self-generated signal. Neurons with smooth processes in the LAL and varicose processes in the OL were present in silkmoth ( Supplementary Fig. 10b for LAL/PS to lobula, 17 for LAL/PS to medulla). GABAergic inhibitory interneurons from premotor to sensory areas, which mediate corollary discharge, have been identified in the mammalian superior colliculus (premotor neurons in the intermediate layer to superficial grey layer) [47] and cerebral cortex (from the secondary motor cortex to auditory cortex) [48] . The similarity existed in the organization of pheromone-processing circuits with other insects. The medial portion of the protocerebrum in fruit fly, Drosophila melanogaster has been shown to receive an input from the subregion in the lateral horn, which receives an input from neurons processing the pheromone [49] , [50] , [51] . The superior protocerebrum was also shown to provide an input to the CX in the fly [52] , [53] , [54] , [55] . The input from the CX in the fly has been reported to converge on the lateral side of the inferior dorsofrontal protocerebra [55] , which roughly corresponds to the upper division of the LAL in the moth. The neurons connecting the SMP and LAL have also been detected in the fly (FlyCircuit; http://www.flycircuit.tw/ [56] ; for example, TH-F-900000 for bilateral, VGlut-F-500768 for a unilateral connection). Putative homologous neurons to other constituents observed in the moth pheromone pathway, such as LAL BNs and DNs, are also present in the fly ( Supplementary Table 2 ). For example, LAL interneurons make contact with the PS and this morphological feature was also observed in the fly ( Supplementary Table 3 ). These results suggest a generality in the circuit design among species. LAL DNs exhibited higher frequencies when the ipsilateral antennae were stimulated ( Fig. 5g ). Differential activation in the early-response phase of DNs may correspond to the initial turning direction [37] . This has also been reported in the reticulospinal cells in lampreys, which showed stronger activity in the side towards which the animal turned than in the opposite side [57] , and the command signal for turning was shown to be encoded by differences in the firing rate between both hemispheres [57] , [58] . The LAL has been considered as the site for the generation of long-lasting activity. We confirmed this long-held assumption by monitoring sensory-evoked activities at all stages of neurons in the present study because (i) neurons did not show long-lasting activity in the SMP, the upstream circuit to the LAL ( Fig. 3i ), and (ii) other types of DNs that did not innervate the LAL also did not show long-lasting activity in response to the sex pheromone. Persistent neural activity is a sustained change in action potential discharge, which outlasts after the sensory input, and has been reported in various neuronal circuits among different animal species [59] . Both single-cell and network mechanisms are thought to be relevant in generating persistent activity. These mechanisms may also be responsible for the long-lasting firing activity in moths. Intrinsic membrane properties that are specific to LAL DNs may contribute to this activity. In the lamprey, transient sensory stimulation induces were shown to induce persistent activity that lasts several minutes at the level of reticulospinal cells, and the local perfusion experiment supports intrinsic cellar mechanisms [60] . Several cellular mechanisms have been proposed for bistability in firing rate (ionic mechanism [61] , [62] ; dendritic spike [63] ). Recurrent synaptic activity in local circuits may also play an important role in generating long-lasting activity, as observed in other systems [64] . For example, persistent activity ceases when synaptic transmission is blocked, suggesting the existence of network mechanisms for transition in ferret neocortex [35] . The crucial role of recurrent excitatory synapses in persistent activity has been reported in the lamprey [65] and zebrafish [66] . Since the phase of the FF neural response correlates among several DNs [14] , the network mechanism may underlie the long-lasting activity observed in moths. The circuit in the lower division of the LAL is a candidate for the mechanism underlying recurrent synaptic activity, because of the longer response duration observed ( Fig. 4e ). Consistent with this, all DNs that exhibited a FF response preferentially innervated the lower LAL ( Supplementary Fig. 15 ). Although such a connection has not yet been reported in insects, an electron microscopic study reports synapses between DNs in the blowfly [67] . Since pure recurrent feedback networks have a robustness problem [59] , we assume that intrinsic membrane properties and circuit recurrent synaptic activity cooperate to generate long-lasting activity in the moth brain, as proposed for persistent activity in other systems. Future work should be directed towards testing the hypothesized contribution of the lower LAL to locomotion by manipulating the neuronal activity. The present study also suggests the circuit homology with D. melanogaster . For example, cell-type-specific manipulation in this genetic model organism enables to investigate the causal role of local circuits within the LAL. The LAL is highly associated with the CX [40] , [55] , which is involved in various aspects of insect behaviour [68] . Descending pathway through the LAL is likely to be common across insects [15] , [16] , [17] , [18] , [31] , [32] , [33] . Our results not only demonstrate an example of a series of neural circuits dedicated for moth olfactory navigation, but also provide insights into the general design of neural circuits for sensory-motor control in insects. Experimental animals B. mori (Lepidoptera: Bombycidae) were reared on an artificial diet (Silk Mate 2S and PS; Nosan Bio Department, Yokohama, Japan) at 26 °C and 60% relative humidity under a long-day photoperiod regime (16/8-h light/dark). Animals were used within 3–7 days of eclosion. Olfactory stimulation Synthetic (E,Z)-10,12-hexadecadien-1-ol (bombykol), the principal pheromone component of B. mori , with a purity of >99%, as confirmed by gas chromatography, was dissolved in HPLC-grade n -hexane. The leaf alcohol cis -3-hexen-1-ol (8.48 μg; H0124, Tokyo Chemical Industries, Japan), a racemic mixture of linalool (8.62 μg; L0048) and citral (8.88 μg; D0762) were also used. The odorant (5-μl solution) was applied to a piece of filter paper (1 × 2 cm) and inserted into a glass stimulant cartridge with a 5.5-mm-tip diameter. The distance between the filter paper and the cartridge exit was ~7 cm. We applied 10 ng of bombykol to the filter paper, which is the amount that induced transient bursting activity in projection neurons in the AL and reliably triggers behavioural responses [69] . Air or the odour stimulus was applied to either side of the antenna, and the exit of the cartridge was positioned 1.5 cm from the antennae. Compressed pure air was passed through a charcoal filter into the stimulant cartridge, and each stimulus was applied at a velocity of 500 ml min −1 (~35 cm s −1 ), nearly the same as the flow speed when moths flap their wings. The moths were exposed to the odour for 200 or 500 ms, after which an exhaust tube was placed on the opposite side of the stimulant cartridge and the odour was removed (inner diameter, 4.5 and 15 cm from the antennae; ~55 cm s −1 ). All stimulant cartridges were sealed with a Teflon sheet, stored at −20 °C, and brought to room temperature prior to the recording session. Single-cell recording and staining with microelectrodes We mainly used intracellular recording technique with glass-sharp microelectrodes for single-cell recording. The recording and staining procedures were conducted as previously described [69] , [70] . Each moth was fixed in a plastic chamber, and its head was immobilized using a notched plastic yoke slipped between the head and the thorax. The brain was exposed by opening the head capsule and removing the large tracheae, and the intracranial muscles were removed to eliminate brain movement. Electrodes with a resistance of ~100–300 MΩ were prepared from thin-walled glass capillaries (TW100F-3 or TW100F-4; World Precision Instruments, Sarasota, FL, USA) using a puller (P-2000 or P-97; Sutter Instruments, Novato, CA, USA). The electrodes were filled with 5% Lucifer yellow CH solution (LY; Sigma, St Louis, MO, USA) in 0.1 M LiCl or 0.1-M potassium chloride to stain the neurons. In some cases, we used juxtacellular recording [9] . Electrodes resembling those used for patch recording were pulled from thin-wall borosilicate glass capillaries and filled with a 4% solution of LY in 0.2 M LiCl, resulting in <30 MΩ electrode resistance. Extracellularly recorded spikes could be distinguished from baseline noise. Recordings including activity from more than one neuron, as judged from spike amplitudes as well as the specificity of responses to pheromone components, were discarded. At the end of a recording period, the preparation was immersed in formaldehyde fixative solution (2.5% formaldehyde in 0.1 M sodium phosphate buffer containing 3% sucrose) with the electrode in place. A silver ground electrode was placed on the head cuticle, and the brain was superfused with saline solution containing 140 mM NaCl, 5 mM KCl, 7 mM CaCl 2 , 1 mM MgCl 2 , 4 mM NaHCO 3 , 5 mM trehalose, 5 mM N-Tris (hydroxymethyl) methyl-2-aminoethanesulfonic acid and 90 mM sucrose (pH 7.3). The electrodes were inserted using a micromanipulator (Leica Microsystems, Wetzlar, Germany), and the incoming signals were amplified (MEZ-8300; Nihon Kohden, Tokyo, Japan), monitored with an oscilloscope (VC-10; Nihon Kohden) and recorded on a DAT recorder (RD-125T; TEAC, Tokyo, Japan) at 24 kHz. The acquired signals were stored in a computer using an A/D converter (PCI-6025E; National Instruments, Austin, TX, USA). Mass staining We performed mass staining under visual control. After cooling to achieve immobility, the brain was dissected from the head capsule. The brain was superfused with physiological saline. We carefully ruptured the sheath over the brain with fine forceps. The brain was placed on a fixed-stage upright microscope (BX50WI; Olympus, Tokyo, Japan) equipped with differential interference contrast optics and long-working-distance objectives ( × 40 LUMPlanFL/IR or × 60 LUMPlanFL/IR water immersion; Olympus). A charge-coupled device camera (C2741-79; Hamamatsu Photonics, Shizuoka, Japan) enhanced contrast. A microelectrode filled with 5% or 10% tetramethylrhodamine dextran (D3308; Molecular Probes, Eugene, OR) or 4% LY solution (L0259, Sigma) was placed in the neuropils. The dye was injected iontophoretically with 5 Hz, 40–100 ms and 0.1–0.7 μA depolarizing current for 5–30 min. We used hyperpolarized current for LY solution. We injected crystals of Texas Red dextran (Molecular Probes) into the PS from the posterior surface of the brain ( Supplementary Fig. 11 ). Glass microelectrodes were broken and dipped into Vaseline to pick up Texas Red dextran crystals. The electrode was then manually inserted into the target area. The superficial tracer was removed by rinsing with saline. The opened area was covered with Vaseline. The preparations were left at 4°C for 1–24 h to allow the dye to diffuse, and the brains were dissected, fixed, dehydrated and cleared as described above. To target the ΔILPC, we inserted the electrode with 50–100 μm from the dorsal side, at the position of 0–100 μm lateral to the AOTu and ±50 μm from the centre of the central body upper division. To target the lateral horn, we inserted the electrode with 50–100 μm from the dorsal side, at the position of 50–150 μm lateral to the AOTu and 0–100 μm posterior to the centre of the central body upper division. To target the SMP, we inserted the electrode from the medio-dorsal side with 50 μm, from 0 to 100 μm posterior to the anterior edge of the MB lobes. To target the LAL, we inserted the electrode with 70–120 μm from the medial side, at the position of 0–50 μm ventral to the ventral edge of the MB medial lobe and 0–100 μm posterior to the anteromost part of the medial lobe. In some cases, we stained multiple neurons with sharp electrodes ( Supplementary Figs 10g–i and 12d ). We repeated intracellular staining at different depths, which were close to each other. All staining sites in the same sample were located within ~30 μm. This operation was able to label multiple neurons running closely with each other. Although the number of stained cells was smaller and the success rate was lower than mass staining with the dye injection mentioned above, this method enabled us to observe the types of neuronal morphology in more detail. Backfill labelling The ventral part of the neck was dissected to expose the neck connective. The nerve was stained by filling with saturated LY dissolved in distilled water from the cut end of the neck connective overnight at 4 °C. The neck connective was placed in the pool made with Vaseline on a cover glass. After backfilling, the head was immediately removed. The brain was dissected from the head, and the brains were dissected, fixed, dehydrated and cleared as described above. Confocal microscopy Confocal images were taken on a Zeiss confocal microscope (LSM510; Carl Zeiss, Jena, Germany) using a × 40 Plan Apochromat 1.0 numerical aperture lens with the following settings: 0.7–1.4 μm z-dimension steps, sequential scanning, 512 × 512 or 1,024 × 1,024 pixels, 12-bit data, scan speed 4 or 5 and bidirectional scanning with auto-z-dimension correction. LY-stained neurons were examined at an excitation wavelength of 458 nm (Argon laser) with a long-pass emission filter (>475 nm) or band-pass filter (505–550 nm) in whole mounts. Tetramethylrhodamine-stained neurons were examined at an excitation wavelength of 543 nm (He-Ne laser) with a long-pass emission filter (>560 nm) in whole mounts. Serial optical sections were acquired at 0.7-μm intervals throughout the entire depth of each neuron. Three-dimensional reconstruction of single neurons Neuron and neuropil tracing was carried out semi-manually using AVIZO 6.3 (Visage Imaging, Carlsbad, CA, USA). After manual tracing, individual objects for neuropils were smoothed using the ‘smooth label’ function. Analysis of neuronal responses Spikes were semi-automatically detected. Responses were divided into 100-ms time bins, and the mean firing rate for each bin was calculated for the peristimulus spike histogram and raster plots. The number of spikes from the stimulus onset to 1 s after was counted as the number of spikes ( Figs 3h and 4d ). The firing rate of the DN response in the early phase was obtained as the rate from the stimulus to 800 ms after ( Fig. 5g ). The response duration was counted as the length when the mean firing rate was higher than the mean+2 s.d. of that in the pre-stimulus period ( Figs 3i and 4e ). Statistical analyses of this distribution were performed using a custom-made program written in MATLAB and statistics toolbox (MathWorks, Natick, MA, USA). All P values for multiple comparisons were calculated by repeated measures analysis of variance. Analysis of neurite distribution The analysis of neurite distribution was basically the same as that described in a previous study [70] . To analyse the distribution of neurites ( Fig. 4 ; Supplementary Figs 5 and 9 ), we calculated the centroids in the volume of the LAL. The anterior surface of the LAL had a clear boundary with the AL. The posterior part of the LAL did not have a clear anatomical boundary with the ventral protocerebrum, and we followed the definition by Iwano et al. [25] , which defined the posterior border of the LAL as the turning point of the lateral antenno-protocerebral tract. Using these coordinates, we aligned the density distribution of each neuron. The neurite distribution of individual LAL BNs was represented as a matrix (10 × 10 × 10 voxels). We defined the areas of the upper and lower divisions of the LAL based on manual segmentation. We obtained the volume for each subdivision by counting the value in corresponding voxels ( Fig. 4 ; Supplementary Figs 5 and 9 ). The relative volume for neurite innervation in each LAL subdivision was obtained as follows: the absolute volume for each division was divided by the volume of the neurite for the anterior portion of the ventral protocerebrum, including the LAL and ventral protocerebrum, but not the PS ( Fig. 4b ). To classify the morphology of LAL BNs, we performed principal component (PC) analysis on 12 LAL BNs. We performed clustering analysis using the first three PCs. High positive values in PC1 and PC2 mostly corresponded to the upper and lower divisions of the LAL. We obtained similar results when we defined LAL subdivisions based on these PCs. The contrast and brightness of images were modified by Image J (National Institutes of Health, Bethesda, MD). Figures were prepared in Adobe Illustrator CS (Adobe systems, San Jose, CA). How to cite this article: Namiki, S. et al. Information flow through neural circuits for pheromone orientation. Nat. Commun. 5:5919 doi: 10.1038/ncomms6919 (2014).